Pore surface engineering in covalent organic frameworks Covalent organic frameworks (COFs) are a class of important porous materials that allow atomically precise integration of building blocks to achieve pre-designable pore size and geometry; however, pore surface engineering in COFs remains challenging. Here we introduce pore surface engineering to COF chemistry, which allows the controlled functionalization of COF pore walls with organic groups. This functionalization is made possible by the use of azide-appended building blocks for the synthesis of COFs with walls to which a designable content of azide units is anchored. The azide units can then undergo a quantitative click reaction with alkynes to produce pore surfaces with desired groups and preferred densities. The diversity of click reactions performed shows that the protocol is compatible with the development of various specific surfaces in COFs. Therefore, this methodology constitutes a step in the pore surface engineering of COFs to realize pre-designed compositions, components and functions. Organic porous frameworks are technologically important materials with myriad functions and applications [1] , [2] , [3] , [4] , [5] , [6] , [7] , [8] , [9] , [10] , [11] , [12] , [13] , [14] . The pore surface forms a microscopic interface with gas or guest molecules, and is an important characteristic that determines the macroscopic nature of these materials in applications such as gas adsorption, molecular separation, catalysis and energy storage. Among these materials, covalent organic frameworks (COFs) are a class of porous materials that feature low-weight elements and strong covalent linkages of their components, and they exhibit high flexibility in their molecular design, which allows the atomically precise integration of their building blocks into porous structures [15] , [16] , [17] , [18] , [19] , [20] , [21] , [22] , [23] , [24] , [25] , [26] , [27] , [28] , [29] , [30] , [31] , [32] , [33] , [34] . COFs can be constructed by the reticular design of their components, which, upon undergoing condensation reactions, form a porous skeleton with a precise pore size and specific pore geometry. Various COFs that possess tetragonal or hexagonal pores in the micro or meso range have been developed by this approach. Despite the availability of a variety of skeletons for COFs, control of the pore surface remains a significant challenge because of difficulties in the development of a strategy that allows systematic engineering of the COF pore walls. Engineering of the pore surface would endow COFs with a tailor-made interface to meet specific application requirements. Synthetic approaches to pore surface control have been reported for non-covalent crystalline metal-organic frameworks (MOFs). An azide-appended MOF exhibits pore surface decoration upon reaction with small alkynes [35] , whereas an MOF bearing trimethylsilane-protected acetylene units allows a selective deprotection and a selective decoration of the exterior and interior surfaces with ethidium bromide and phenyl groups, respectively, by reaction with the corresponding azide compounds [36] . Despite these achievements, density control of the functional surface groups in MOFs has not been obtained. Furthermore, COFs with long alkyl chains and large groups appended on the walls are difficult to prepare by direct condensation reactions. Here we report our strategy for the pore surface engineering of COFs. Our strategy offers precise control over the composition, density and functionalities of organic groups anchored onto the pore walls. For this purpose, an azide-appended phenylene block was synthesized and utilized as the wall component in a two-component condensation system for the construction of COFs with azide-integrated walls. The two-component system was further developed to a three-component system that consists of azide-appended phenylene, 'naked' phenylene walls and corner blocks, thereby enabling the synthesis of COFs that bear a tuneable amount of azide units on the walls. The azide units on the COF walls were found to undergo a quantitative click reaction with alkynes to form triazole-linked groups on the wall surfaces. Consequently, the combination of a three-component condensation system with the click reaction resulted in the establishment of a protocol that allows the control of both the composition and density of organic groups in the pores. This methodology is demonstrated to be widely useful for the creation of various specific surfaces in COF pores. Azide-appended COFs COF-5 is a typical mesoporous COF that consists of triphenylene at the corners and phenylene on the walls of a boronate ester-linked two-dimensional (2D) hexagonal skeleton [15] . We introduced azide groups to the 2 and 5 positions of the phenylene unit of 1,4-benzenediboronic acid, and utilized the azide-appended benzenediboronic acid (N 3 -BDBA) as wall blocks for the condensation reaction with hexahydroxytriphenylene (HHTP) ( Fig. 1 ). The resulting hexagonal skeleton is identical to that of COF-5, with triphenylene corners but azide-appended phenylene walls. This strategy allows the growth of various specific groups on the surface because the azide units in the skeletons are reactive groups that can click with various alkynes for pre-designable functionalization. The condensation reaction of N 3 -BDBA and HHTP was performed in a mixed solvent of 1,4-dioxane and mesitylene at 80°C for 3 days and afforded a light-yellow precipitate. The precipitate was washed five times with anhydrous acetone and then dried under vacuum to provide 100%N 3 -COF-5 in 72% isolated yield. The yield of the condensation reaction was similar to that for COF-5. 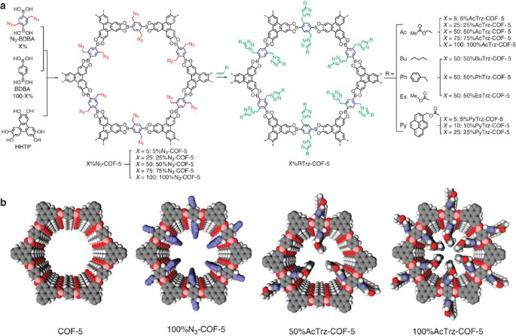Figure 1: Pore surface engineering in COFs. (a) The scheme shows a general strategy for the surface engineering of COFs through the combination of condensation reaction and click chemistry. In the first step, COFs bearing azide units on the walls are synthesized by the condensation reaction of HHTP with azide-appended benzene diboronic acid (N3-BDBA) and benzene diboronic acid (BDBA) in a designated molar ratio (X=0–100%). The content of N3-appended wall units is tunable from 0 to 100%, depending on the molar ratio of N3-BDBA to BDBA. Five members of X%N3-COF-5 with different contents (X=5, 25, 50, 75 and 100) were synthesized. The structure of 100%N3-COF-5 was shown in the figure, with all of the walls occupied by the N3-appended phenylene units. In the next step, the azide groups on the COF walls are clicked with alkynes to anchor various organic groups onto the walls of COFs (X%RTrz-COF-5). The density of R surface groups on the walls is determined by the azide content in X%N3-COF-5. (b) Graphical representation of COF-5 upon surface engineering, which leads to the functionalization of organic groups on the walls. The component, composition and density of the organic groups on the walls are controllable. Figure 1: Pore surface engineering in COFs. ( a ) The scheme shows a general strategy for the surface engineering of COFs through the combination of condensation reaction and click chemistry. In the first step, COFs bearing azide units on the walls are synthesized by the condensation reaction of HHTP with azide-appended benzene diboronic acid (N 3 -BDBA) and benzene diboronic acid (BDBA) in a designated molar ratio ( X =0–100%). The content of N 3 -appended wall units is tunable from 0 to 100%, depending on the molar ratio of N 3 -BDBA to BDBA. Five members of X%N 3 -COF-5 with different contents ( X =5, 25, 50, 75 and 100) were synthesized. The structure of 100%N 3 -COF-5 was shown in the figure, with all of the walls occupied by the N 3 -appended phenylene units. In the next step, the azide groups on the COF walls are clicked with alkynes to anchor various organic groups onto the walls of COFs (X%RTrz-COF-5). The density of R surface groups on the walls is determined by the azide content in X%N 3 -COF-5. ( b ) Graphical representation of COF-5 upon surface engineering, which leads to the functionalization of organic groups on the walls. The component, composition and density of the organic groups on the walls are controllable. Full size image The azide units were retained well without decomposition during the condensation reaction. Elemental analysis of 100%N 3 -COF-5 revealed that the nitrogen content was 20.0%, which is close to the calculated value of 17.7% for an infinite 2D skeleton ( Supplementary Table S1 ). Infrared (IR) spectroscopy provided direct evidence for the presence of azide units with a typical vibration band at 2,102 cm –1 , which was absent in the case of COF-5 ( Fig. 2 , green and dotted black curves). On the other hand, 100%N 3 -COF-5 displayed vibration bands arising from boronate ester linkages, which connect the wall and corner blocks, at 1,074, 1,160, 1,244 and 1,308 cm –1 ; these bands were identical to those observed for COF-5 ( Fig. 2 , filled circles). 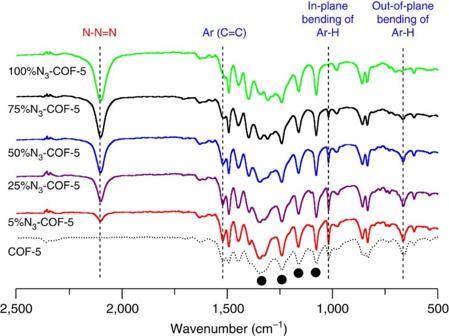Figure 2: IR spectral profiles. IR spectra displayed characteristic vibration bands due to the azide and phenylene groups of azide-anchored COF-5. The N3signal was absent in COF-5 and increased in intensity for X%N3-COF-5 when the N3-appended wall content was increased. On the other hand, signals for the C=C and Ar–H units of the phenylene edges decreased with the N3-appended phenylene content. The vibration bands due to boronate ester linkages are the same as those of COF-5, as indicated with filled circles. Figure 2: IR spectral profiles. IR spectra displayed characteristic vibration bands due to the azide and phenylene groups of azide-anchored COF-5. The N 3 signal was absent in COF-5 and increased in intensity for X%N 3 -COF-5 when the N 3 -appended wall content was increased. On the other hand, signals for the C=C and Ar–H units of the phenylene edges decreased with the N 3 -appended phenylene content. The vibration bands due to boronate ester linkages are the same as those of COF-5, as indicated with filled circles. Full size image X-ray diffraction (XRD) measurements revealed that 100%N 3 -COF-5 produced a strong peak at 2 θ =3.48° together with relatively weak signals at 5.99, 6.96, 9.18 and 26.24° ( Fig. 3a , green curve), which were assigned to the 100, 110, 200, 300 and 001 facets, respectively. The 2 θ values and linewidths of these XRD peaks were almost identical to those for COF-5 ( Fig. 3a , black curve). The Pawley refined pattern ( Fig. 3b , blue curve) confirmed the XRD peak assignments, as the difference from the observed XRD pattern was negligible ( Fig. 3b , black curve). A geometric optimization showed that the azide units were extended in the same plane of the 2D polymer skeleton. Simulations based on the XRD pattern using an AA stacking structure of the P 6/ m (175) space group ( Supplementary Table S2 ) with a = b =30.010 Å, c =3.450 Å and α = β =90°, γ =120° resulted in an XRD pattern that was in good agreement with the experimentally observed pattern ( Fig. 3b , blue curve). In this formulation, the centre-to-centre pore distance is 3.0 nm in the 2D plane, and the 2D sheets stack to form layers separated by a distance of 3.4 Å. 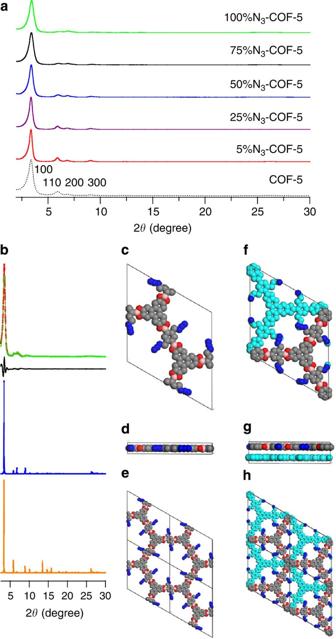Figure 3: XRD patterns and crystalline structure. (a) XRD patterns of X%N3-COF-5 (X=5, 25, 50, 75 and 100) and COF-5. The diffraction peaks from 100, 110, 200, 300 and 001 facets of X%N3-COF-5 are the same as those for COF-5. The introduction of azide units to the phenylene walls does not affect the AA stacking structure of COFs. (b) XRD pattern simulation of 100%N3-COF-5. The green curve is experimentally observed XRD pattern, red curve is Pawley refinement and black curve is their difference. The blue curve is the simulated XRD pattern based on the AA stacking model (P6/m) and orange curve is that based on the AB stacking model (P63mc). The AA stacking model reproduces the experimental XRD pattern, while the AB stacking model cannot reproduce the XRD pattern. (c) The unit-cell structure of 100%N3-COF-5 derived using the AA stacking model alongzaxis. (d) The unit-cell structure of the AA stacking alongyaxis. (e) A single pore structure. (f) The unit-cell structure using staggered AB stacking model alongzaxis. (g) The unit-cell structure of the AB stacking alongyaxis. (h) A staggered pore structure. Figure 3c–e shows the derived unit-cell structure. In contrast, a staggered AB stacking arrangement of the layers from the P 6 3 mc space group (186) did not reproduce the experimental XRD pattern ( Fig. 3b , orange curve). Figure 3f,g shows the unit cell for the AB-type staggered stacking arrangement. In this arrangement, the 2D sheet overlaps on the pores of the neighbouring sheet ( Fig. 3h ). Figure 3: XRD patterns and crystalline structure. ( a ) XRD patterns of X%N 3 -COF-5 ( X =5, 25, 50, 75 and 100) and COF-5. The diffraction peaks from 100, 110, 200, 300 and 001 facets of X%N 3 -COF-5 are the same as those for COF-5. The introduction of azide units to the phenylene walls does not affect the AA stacking structure of COFs. ( b ) XRD pattern simulation of 100%N 3 -COF-5. The green curve is experimentally observed XRD pattern, red curve is Pawley refinement and black curve is their difference. The blue curve is the simulated XRD pattern based on the AA stacking model ( P 6/ m ) and orange curve is that based on the AB stacking model ( P 6 3 mc ). The AA stacking model reproduces the experimental XRD pattern, while the AB stacking model cannot reproduce the XRD pattern. ( c ) The unit-cell structure of 100%N 3 -COF-5 derived using the AA stacking model along z axis. ( d ) The unit-cell structure of the AA stacking along y axis. ( e ) A single pore structure. ( f ) The unit-cell structure using staggered AB stacking model along z axis. ( g ) The unit-cell structure of the AB stacking along y axis. ( h ) A staggered pore structure. Full size image The content of azide units on the pore walls can be tuned using a three-component condensation system with HHTP as the corners and a mixture of N 3 -BDBA and BDBA as the walls. As shown in the two-component system, the azide units in N 3 -BDBA did not affect the reactivity of BDBA in the condensation reaction. Therefore, changing the ratio of N 3 -BDBA to BDBA permits the regulation of the overall azide content on the walls. To demonstrate this property, an equimolar mixture of N 3 -BDBA and BDBA was employed for the condensation reaction with HHTP under conditions identical to those used for 100%N 3 -COF-5. The condensation reaction yielded 50%N 3 -COF-5 with an azide-appended phenylene edge content that was calculated to be ~50% based on the elemental analysis. The coexistence of azide-appended phenylene units and 'naked' phenylene walls was further confirmed by IR spectroscopy, with vibration bands displayed at 2,102 cm –1 for the azide unit, at 1,520 cm –1 for the phenyl C=C bond and at 1,021 cm –1 (in-plane bending) and 662 cm –1 (out-of-plane bending) for the phenyl C–H bond ( Fig. 2 , blue curve). The XRD profile for 50%N 3 -COF-5 was similar to that for 100%N 3 -COF-5 ( Fig. 3 , blue curve), which indicates the retention of the crystalline structure. The three-component system can be further extended to the synthesis of COFs with desired contents of azide units. This concept was confirmed by condensation reactions using different N 3 -BDBA contents at molar ratios of 5, 25 and 75% relative to BDBA. Interestingly, these reactions provided the corresponding 5%N 3 -COF-5, 25%N 3 -COF-5 and 75%N 3 -COF-5, respectively, that bore the designated azide contents as evaluated by elemental analysis ( Supplementary Table S1 ), thermogravimetric analysis (TGA) and IR spectroscopy. TGA analyses of the X%N 3 -COF-5 samples revealed a weight loss at 270°C that was attributed to the azide units, and the percentage weight losses were identical to the azide unit contents in X%N 3 -COF-5 ( Supplementary Fig. S1 ). IR spectra showed that as the azide unit content in the COFs increased, the intensity of the vibration band attributed to the azide units (2,102 cm –1 ) increased, whereas those attributed to the phenyl C=C and C–H bonds decreased accordingly ( Fig. 2 ). XRD measurements revealed that all the azide-anchored COFs produced identical diffraction patterns, which indicates that they had the same crystalline stacking model as 100%N 3 -COF-5, irrespective of the azide unit content on the walls ( Fig. 3 ; Supplementary Fig. S2 ). The decrease in the relative intensity of the XRD peaks observed for 75%N 3 -COF-5 and 100%N 3 -COF-5 is related to the high content of rotatable benzyl azide units, as has been reported for alkyl-appended COFs [19] . Nitrogen sorption isotherm measurements were obtained to characterize the porous structures of X%N 3 -COF-5. All of the X%N 3 -COF-5 samples exhibited typical type-IV sorption isotherm profiles that are indicative of the mesoporous character ( Fig. 4a ). Table 1 summarizes the regulation of the pore surface area, volume and size according to the azide content. As the content of azide-appended walls was increased, the Brunauer–Emmett–Teller (BET) surface area, pore volume and pore size decreased. These changes are attributed to the decrease in the volume of the pores that are accessible to nitrogen gas because the space occupied by the azide units increases with their content ( Fig. 1b ). Pore size distribution profiles for X%N 3 -COF-5 revealed that the azide-appended COFs predominantly possess single mesopores, which accounts for the high surface areas of these COFs ( Fig. 4b ). Therefore, the three-component condensation systems allow the integration of azide-appended walls into COFs in a controlled manner with retention of the crystalline and porous structure. 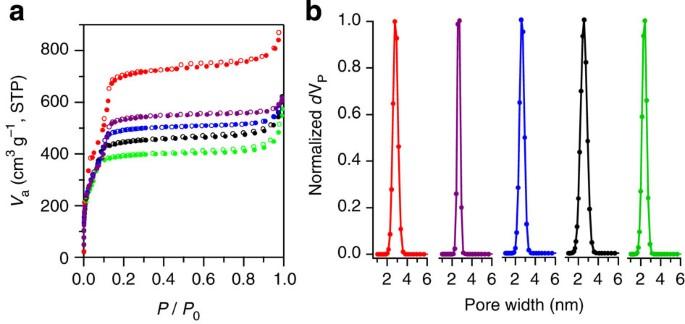Figure 4: Porous structures. (a) N2sorption isotherm profiles of X%N3-COF-5 reveal typical type-IV sorption curves, which are indicative of mesoporous characters (red: 5%N3-COF-5; purple: 25%N3-COF-5; blue: 50%N3-COF-5; black: 75%N3-COF-5; green: 100%N3-COF-5). The filled circle is adsorption and open circle is desorption process, respectively. (b) Pore size distribution profiles of X%N3-COF-5 exhibit single mesopore for all of the X%N3-COF-5 samples (colours represent the same COFs as indicated ina). Figure 4: Porous structures. ( a ) N 2 sorption isotherm profiles of X%N 3 -COF-5 reveal typical type-IV sorption curves, which are indicative of mesoporous characters (red: 5%N 3 -COF-5; purple: 25%N 3 -COF-5; blue: 50%N 3 -COF-5; black: 75%N 3 -COF-5; green: 100%N 3 -COF-5). The filled circle is adsorption and open circle is desorption process, respectively. ( b ) Pore size distribution profiles of X%N 3 -COF-5 exhibit single mesopore for all of the X%N 3 -COF-5 samples (colours represent the same COFs as indicated in a ). Full size image Table 1 Pore parameters of azide and acetyl functionalized COF-5. Full size table Pore surface engineering with acetyl units Azide units are well established for click reactions with alkynes to introduce functional groups via 1,2,3-triazole rings (Trz) [37] . We investigated the reactivity of azide units on the walls of X%N 3 -COF-5 ( X =5, 25, 50, 75 and 100) in a typical click reaction with 2-propynyl acetate in anhydrous N , N -dimethylacetamide (DMAc) at 50°C with CuI present as a catalyst. After the reaction was allowed to proceed for 24 h, the precipitates were collected using a centrifuge, and washed with excess anhydrous DMAc and acetone to provide the corresponding X%AcTrz-COF-5 in quantitative yields. TGA revealed that the weight loss attributed to the surface groups on the pore walls was identical to the content of these groups in X%AcTrz-COF-5 ( Supplementary Fig. S3 ). The typical vibration band at 2,102 cm –1 , which was assigned to the azide units, disappeared for all X%N 3 -COF-5 samples, irrespective of the azide unit content ( Fig. 5a ); this disappearance indicates the completion of the click reactions in each case. In addition, a new C=O vibration band that corresponded to the acetyl units appeared at 1,730 cm –1 and increased almost linearly in intensity with the acetyl unit content in X%AcTrz-COF-5 ( Fig. 5a ). XRD measurements revealed almost no change in the 2 θ values for all X%AcTrz-COF-5 samples compared with the X%N 3 -COF-5 samples, which confirms that the AA stacking structure of the COF skeletons was retained ( Fig. 5b ). A decrease in the intensity and a broadening of the XRD peak linewidths were observed for the 75%AcTrz-COF-5 and 100%AcTrz-COF-5 samples because of the high density of the flexible acetyl termini with amorphous character ( Fig. 5 and Supplementary Fig. S4 ), which is coincident with the tendency reported for alkyl-appended COFs [18] . These results indicate that the acetyl units are anchored via a triazole linkage onto the walls of COFs such that the position and contents are identical to those of the precursor azide-anchored COFs. Therefore, the strategy of a three-component condensation system combined with click reactions not only leads to the formation of organic surface groups in COFs, but also allows the tuning of the density of these groups on the pore walls. 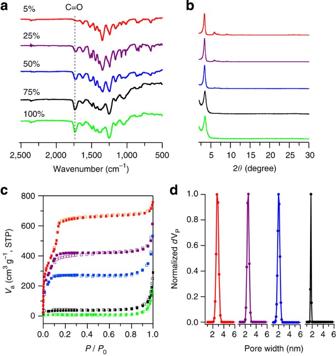Figure 5: COFs engineered with acetyl surface. (a) IR spectra of X%AcTrz-COF-5 (X=5, 25, 50, 75 and 100%) after click reaction of X%N3-COF-5 with 2-propynyl acetate. The characteristic vibration band due to the N3groups disappeared, while new vibration bands due to the carboxyl groups appeared. (b) XRD profiles of X%AcTrz-COF-5. The XRD patterns are similar, which indicate that the stacking models were well retained for these COFs. (c) Nitrogen sorption isotherm profiles of X%AcTrz-COF-5. (d) Pore size distribution profiles of X%N3-COF-5 exhibited solely single pores for X%AcTrz -COF-5. When X increased, the pore changed from mesopores to micropores. The colours of curves represent the same COFs as indicated ina. Figure 5: COFs engineered with acetyl surface. ( a ) IR spectra of X%AcTrz-COF-5 ( X =5, 25, 50, 75 and 100%) after click reaction of X%N 3 -COF-5 with 2-propynyl acetate. The characteristic vibration band due to the N 3 groups disappeared, while new vibration bands due to the carboxyl groups appeared. ( b ) XRD profiles of X%AcTrz-COF-5. The XRD patterns are similar, which indicate that the stacking models were well retained for these COFs. ( c ) Nitrogen sorption isotherm profiles of X%AcTrz-COF-5. ( d ) Pore size distribution profiles of X%N 3 -COF-5 exhibited solely single pores for X%AcTrz -COF-5. When X increased, the pore changed from mesopores to micropores. The colours of curves represent the same COFs as indicated in a . Full size image The X%AcTrz-COF-5 samples exhibited reversible nitrogen sorption isotherms; however, the profiles were highly dependent on the density of surface groups on the pore walls ( Fig. 5c ). The 5%AcTrz-COF-5 and 25%AcTrz-CFO-5 exhibited typical type-IV curves ( Fig. 5c , red and purple curves), which are characteristic of the mesoporous character. However, 50%AcTrz-CFO-5, 75%AcTrz-CFO-5 and 100%AcTrz-CFO-5 displayed typical microporous sorption curves ( Fig. 5c ). As shown in Table 1 , the content of the surface groups on the walls allows the regulation of the BET surface area, pore volume and pore size. A sharp decrease in the BET surface area and pore volume was observed for 75%AcTrz-CFO-5 and 100%AcTrz-CFO-5 ( Table 1 ). Considered together with the significantly weakened XRD signals of the 001 facets for 75%AcTrz-COF-5 and 100%AcTrz-COF-5, these results suggest that the stacked layers in75%AcTrz-COF-5 and 100%AcTrz-COF-5 are probably de-lamellate. The dense surface units anchored on the walls endow the COFs with increased solubility. The pore size distribution profiles reveal that the porosity is predominately derived from the solely micro- or mesopores of X%AcTrz-COF-5, which indicates that the pore walls are homogeneously functionalized ( Fig. 5d ). Pore surface engineering allows control of the pore size, which can be precisely regulated from the mesoporous down to the microporous scale, depending on the density of the surface groups ( Table 1 ). For example, 5%AcTrz-COF-5 and 25%AcTrz-COF-5 possess mesopores with sizes of 3.0 and 2.4 nm, respectively, whereas 75%AcTrz-COF-5 and 100%AcTrz-COF-5 are supermicroporous and exhibit pore sizes of 1.6 and 1.2 nm, respectively. The present strategy can be further extended to the introduction of various specific groups onto the walls of COFs. To demonstrate this property, we selected a paraffinic unit, an aromatic hydrocarbon and ester groups as typical examples, and selected 50%N 3 -COF-5 as a platform for the click reaction because of its moderate azide content and high crystallinity. Click reactions of 50%N 3 -COF-5 with 1-hexyne, 3-phenyl-1-propyne and methyl propiolate were quantitatively achieved, and led to the integration of n -butyl, benzyl and methyl ester units to the termini of the triazole groups to provide 50%BuTrz-COF-5, 50%PhTrz-COF-5 and 50%EsTrz-COF-5, respectively. IR spectroscopy confirmed the completion of the click reactions ( Fig. 6a , red, purple and blue curves), and XRD measurements revealed the retention of the AA stacking model in all of the COFs ( Fig. 6b , red, purple and blue curves). The 50%BuTrz-COF-5 ( Fig. 6c , red curve), 50%PhTrz-COF-5 (purple curve) and 50%EsTrz-COF-5 (blue curve) exhibited similar nitrogen sorption isotherm curves and displayed mesoporous characteristics. The BET surface area, pore volume and pore size of these COFs were evaluated as 1,080, 1,001 and 996 m 2 g –1 ; 1.032, 0.809 and 0.684 cm 3 g −1 ; and 2.322, 2.125 and 2.132 nm, respectively ( Supplementary Table S3 ). The pore size distribution profiles indicate that single pores are present in the COFs, which accounts for the porosity of the resulting COFs after the click reactions ( Supplementary Fig. S5 ). A further demonstration of the versatility of this click reaction approach was conducted for the integration of π-electronic components onto the walls. A typical chromophore, that is, pyrene, was selected as a fluorescent tag to label the walls. Click reactions of 5%N 3 -COF-5 with (3 α 1 , 3 α 2 -dihydropyren-1-yl)methyl propionate (PyMP) quantitatively yielded 5%PyTrz-COF-5. The effective introduction of pyrene units to the walls was revealed by the absence of the azide vibration band (2,102 cm –1 ) and the appearance of the C=O vibration band (1,718 cm –1 ) in the IR spectra ( Fig. 6a , black curve). XRD measurements confirmed that the crystalline structure of 5%PyTrz-COF-5 was well retained ( Fig. 6b , black curve). The 5%PyTrz-COF-5 exhibited a mesoporous character in the nitrogen sorption isotherm profiles and a BET surface area of 1,906 m 2 g –1 ( Fig. 6c , black curve). Under identical conditions, the reaction of PyMP with 10%N 3 -COF-5 and 25%N 3 -COF-5 provided the corresponding 10%PyTrz-COF-5 and 25%PyTrz-COF-5, respectively, with corresponding XRD patterns and nitrogen sorption isotherm profiles ( Fig. 6a–d ). Although azide-appended COF-5 is not fluorescent, the anchoring of pyrene chromophores on the walls allows the COF to fluoresce; 5%PyTrz-COF-5 provided a brilliant blue emission at 450 nm upon excitation of the pyrene unit at 351 nm ( Fig. 6d , black curve; Supplementary Fig. S6 ). When the pyrene content was increased, a red shift of the emission band to 464 nm was observed (25%PyTrz-COF-5, Fig. 6d , orange curve). In contrast, the monomeric PyMP displayed an excimer emission at 475 nm in the solid state ( Fig. 6d , dotted black curve). However, when pyrene units are utilized as the edge unit of COFs (TP-COF and PPy-COF), the eclipsed stacking of pyrene edges eventually leads to typical excimer emissions at 474 and 484 nm [21] , [25] . The blue shifts of the emission band observed for 25%PyTrz-COF-5 with respect to PyMP, TP-COF and PPy-COF suggest that the excimer formation of pyrene units is weakened. Therefore, the pore walls of COFs serve as a 'molecular partition' and provide a scaffold that can prevent chromophores from aggregation. 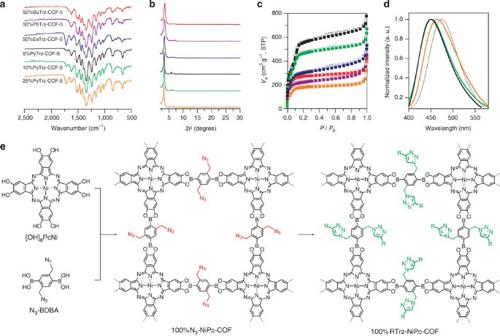Figure 6: COFs engineered with various organic groups. (a) IR spectra of 50%BuTrz-COF-5 (red curve), 50%PhTrz-COF-5 (purple curve) and 50%EsTrz-COF-5 (blue curve), synthesized by the click reaction of 50%N3-COF-5 with 1-hexyne, 3-phenyl-1-propyne and methyl propiolate, respectively, to introduce paraffin chain, aromatic ring and ester groups to the surface of the pores. Black, green and orange curves correspond to 5%PyTrz-COF-5, 10%PyTrz-COF-5 and 25%PyTrz-COF-5, respectively, with pyrene fluorescent tags labelled on the wall. The azide vibration band disappeared. Instead, new vibration bands due to the carboxyl, phenyl and alkyl groups appeared. (b) XRD profiles of 50%BuTrz-COF-5 (red curve), 50%PhTrz-COF-5 (purple curve), 50%EsTrz-COF-5 (blue curve), 5%PyTrz-COF-5 (black curve), 10%PyTrz-COF-5 (green curve) and 25%PyTrz-COF-5 (orange curve) are similar, which indicated that the stacking models were well retained for COFs engineered with different surface. (c) Nitrogen sorption isotherm profiles revealed that 50%BuTrz-COF-5 (red curve), 50%PhTrz-COF-5 (purple curve), 50%EsTrz-COF-5 (blue curve), 5%PyTrz-COF-5 (black curve) and 10%PyTrz-COF-5 (green curve) are mesoporous, while 25%PyTrz-COF-5 (orange curve) is microporous. (d) Fluorescence profiles of 5%PyTrz-COF-5 (black curve), 10%PyTrz-COF-5 (green curve) and 25%PyTrz-COF-5 (orange curve) revealed blue-shifted emission with respect to monomeric pyrene (dotted black curve). (e) Schematic representation of the surface engineering of the typical tetragonal NiPc-COF. The NiPc-COF walls can be engineered as demonstrated by 100%RTrz-COF (R=Es). Figure 6: COFs engineered with various organic groups. ( a ) IR spectra of 50%BuTrz-COF-5 (red curve), 50%PhTrz-COF-5 (purple curve) and 50%EsTrz-COF-5 (blue curve), synthesized by the click reaction of 50%N 3 -COF-5 with 1-hexyne, 3-phenyl-1-propyne and methyl propiolate, respectively, to introduce paraffin chain, aromatic ring and ester groups to the surface of the pores. Black, green and orange curves correspond to 5%PyTrz-COF-5, 10%PyTrz-COF-5 and 25%PyTrz-COF-5, respectively, with pyrene fluorescent tags labelled on the wall. The azide vibration band disappeared. Instead, new vibration bands due to the carboxyl, phenyl and alkyl groups appeared. ( b ) XRD profiles of 50%BuTrz-COF-5 (red curve), 50%PhTrz-COF-5 (purple curve), 50%EsTrz-COF-5 (blue curve), 5%PyTrz-COF-5 (black curve), 10%PyTrz-COF-5 (green curve) and 25%PyTrz-COF-5 (orange curve) are similar, which indicated that the stacking models were well retained for COFs engineered with different surface. ( c ) Nitrogen sorption isotherm profiles revealed that 50%BuTrz-COF-5 (red curve), 50%PhTrz-COF-5 (purple curve), 50%EsTrz-COF-5 (blue curve), 5%PyTrz-COF-5 (black curve) and 10%PyTrz-COF-5 (green curve) are mesoporous, while 25%PyTrz-COF-5 (orange curve) is microporous. ( d ) Fluorescence profiles of 5%PyTrz-COF-5 (black curve), 10%PyTrz-COF-5 (green curve) and 25%PyTrz-COF-5 (orange curve) revealed blue-shifted emission with respect to monomeric pyrene (dotted black curve). ( e ) Schematic representation of the surface engineering of the typical tetragonal NiPc-COF. The NiPc-COF walls can be engineered as demonstrated by 100%RTrz-COF (R=Es). Full size image The present strategy can be useful for the surface engineering of other COFs. The same protocol was applied to a typical tetragonal mesoporous metallophthalocyanine COF, that is, NiPc-COF ( Fig. 6e ) [30] . Condensation of [OH] 8 PcNi with N 3 -BDBA in a mixture of o -dichlorobenzene and DMAc at 85°C resulted in 100%N 3 -NiPc-COF with a 75% yield. The formation of 100%N 3 -NiPc-COF was supported by various spectroscopic measurements ( Supplementary Fig. S7 , IR spectrum). The azide units did not affect the stacking model of NiPc-COF, as evidenced by the XRD pattern, which was the same as that of NiPc-COF ( Supplementary Fig. S8 ). Nitrogen sorption isotherm measurements revealed that 100%N 3 -NiPc-COF is a microporous COF with a BET surface area of 675 m 2 g –1 ( Supplementary Fig. S9 ), which is similar to the BET surface area of NiPc-COF (624 m 2 g –1 ) [29] . The pore size was evaluated as 1.77 nm ( Supplementary Fig. S10 ), which is smaller than that of NiPc-COF (2.2 nm). The azide surface of 100%N 3 -NiPc-COF can undergo a click reaction for the development of specific surface groups on the pore walls of NiPc-COF ( Fig. 6e ). For example, the click reaction with methyl propiolate leads to the quantitative formation of 100%EsTrz-NiPc-COF with an engineered methyl ester surface on the walls, as evidenced by IR spectroscopy, XRD and nitrogen sorption isotherm measurements ( Supplementary Figs S7-S10 ). Therefore, the pore walls of NiPc-COF could also be engineered with the same method used for the pore walls of COF-5. As shown in above, pore surface engineering results in a drastic change in the pore size, shape and microenvironment. Furthermore, the different functional groups on the pore walls would have a different affinity to gas molecules. The COF-5 frameworks upon surface engineering with different groups at different densities would display a different adsorption capability for different gas molecules and may have a high probability of selective adsorption. To demonstrate this property, we focused on the selective sorption of CO 2 over N 2 , which is a challenging subject in relation to the global warming issue. The gas-sorption selectivity of CO 2 over N 2 for the surface-engineered COF-5 was investigated in comparison with that for COF-5. As shown in Supplementary Figure S11 , the normalized selectivity of the surface-engineered COF-5 depends significantly on the surface groups. The X%PyTrz-COF-5 exhibited an increased tendency for selectivity with increasing pyrene content, and 25%PyTrz-COF-5 exhibited a fivefold increased selectivity in comparison with COF-5. The 50%BuTrz-COF-5, 50%EsTrz-COF-5 and 50%PhTrz-COF-5 displayed selectivities of 2.3, 1.1 and 1.6, respectively. Most significantly, 100%AcTrz-COF-5 showed a 16-fold increase in selectivity relative to that of COF-5. These results indicate that the pore surface is an important factor that affects the sorption properties of the COFs. The tailor-made surface engineering with acidic groups, basic groups and other specific functionalities that interact with target gases or molecules has a high probability of achieving high capacity and selectivity. In this context, the present approach offers numerous possibilities for gas storage and separation. In summary, the present strategy for the pore surface engineering of COFs is simple and universal. This approach enables high throughput because of its highly efficient condensation reaction and the quantitative click reactions. Surface engineering thus offers a synthetic pathway to COFs with long chains or large groups on the surface that cannot be synthesized by a direct condensation reaction. The most significant feature is that the combination of condensation and click reactions enables the molecular design of pore surfaces with controlled composition, components and density. Therefore, this approach provides a new aspect in the chemistry of these well-defined porous materials, and provides a means to tailor pores for specific purposes and applications. Materials 1,4-Dibromo-2,5-dimethylbenzene (Tokyo Kasei Kogyo Co., >98%), tert-butyllithium (Kanto Chemical Co., 1.7 M in pentane solution), 2-isopropoxy-4,4,5,5- tetramethyl-1,3,2-dioxaborolane (Tokyo Kasei Kogyo Co., >98%), N-bromosuccimide (Tokyo Kasei Kogyo Co., >98%), dibenzyl peroxide (Aldrich Chemical Co., >75%) and sodium azide (Tokyo Kasei Kogyo Co., >98%) were used as received. THF was distiled over sodium under Ar before use. Anhydrous DMAc (Kanto Chemical Co., >99%) and anhydrous acetone (Wako Pure Chemical Int., >99%) solvents were used as received. Other reagents were used as received without further purification. N 3 -BDBA and PyMP were synthesized according to the method as shown in Supplementary Methods . Synthesis of 100%N 3 -COF-5 A 1,4-dioxane/mesitylene (2 ml/2 ml in volume) mixture of 2,5-bis(azidomethyl)benzene-1,4-diboronic acid (N 3 -BDBA) (55.2 mg, 0.2 mmol) and HHTP (43.2 mg, 0.133 mmol) in a 10-ml Pyrex tube was degassed via three freeze–pump–thaw cycles. The tube was sealed and heated at 80°C for 3 days. The resulting precipitate was collected by centrifugation, washed with anhydrous acetone (6 ml×5), and dried at 80°C under vacuum, to produce 100%N 3 -COF-5 as a light-yellow solid in 72% isolated yield. Synthesis of 75%N 3 -COF-5 A 1,4-dioxane/mesitylene (2 ml/2 ml in volume) mixture of N 3 -BDBA (41.4 mg, 0.15 mmol), benzene-1,4-diboronic acid (BDBA) (8.3 mg, 0.05 mmol) and HHTP (43.2 mg, 0.133 mmol) in a 10-ml Pyrex tube was degassed via three freeze–pump–thaw cycles. The tube was sealed and heated at 80 °C for 3 days. The resulting precipitate was collected by centrifugation, washed with anhydrous acetone (6 ml×5), and dried at 80°C under vacuum, to produce 75%N 3 -COF-5 as a light-yellow solid in 73% isolated yield. Synthesis of 50%N 3 -COF-5 A 1,4-dioxane/mesitylene (2 ml/2 ml in volume) mixture of N 3 -BDBA (27.6 mg, 0.1 mmol), BDBA (16.6 mg, 0.1 mmol) and HHTP (43.2 mg, 0.133 mmol) in a 10-ml Pyrex tube was degassed via three freeze–pump–thaw cycles. The tube was sealed and heated at 80°C for 3 days. The resulting precipitate was collected by centrifugation, washed with anhydrous acetone (6 ml×5), and dried at 80°C under vacuum, to produce 50%N 3 -COF-5 as a light-yellow solid in 73% isolated yield. Synthesis of 25%N 3 -COF-5 A 1,4-dioxane/mesitylene (2 ml/2 ml in volume) mixture of N 3 -BDBA (13.8 mg, 0.05 mmol), BDBA (24.9 mg, 0.15 mmol) and HHTP (43.2 mg, 0.133 mmol) in a 10-ml Pyrex tube was degassed via three freeze–pump–thaw cycles. The tube was sealed and heated at 80 °C for 3 days. The resulting precipitate was collected by centrifugation, washed with anhydrous acetone (6 ml×5), and dried at 80°C under vacuum, to produce 25%N 3 -COF-5 as a light-yellow solid in 74% yield. Synthesis of 5%N 3 -COF-5 A 1,4-dioxane/mesitylene (2 ml/2 ml in volume) mixture of N 3 -BDBA (2.8 mg, 0.01 mmol), BDBA (31.5 mg, 0.19 mmol) and HHTP (43.2 mg, 0.133 mmol) in a 10-mL Pyrex tube was degassed via three freeze–pump–thaw cycles. The tube was sealed and heated at 80°C for 3 days. The resulting precipitate was collected by centrifugation, washed with anhydrous acetone (6 ml×5), and dried at 80°C under vacuum, to produce 25%N 3 -COF-5 as a light-yellow solid in 71% yield. Click reaction of X%N 3 -COF-5 with 2-propynyl acetate 2-Propynyl acetate (400 μl, 4.03 mmol) was added to a mixture of X%N 3 -COF-5 ( X =5, 25, 50, 75 and 100) (10 mg) and CuI (1.0 mg) in dry DMAc (1.0 ml) in Pyrex tube. The tube was degassed via three freeze–pump–thaw cycles, and the mixture was stirred at 50°C for 24 h. The precipitate was collected by centrifugation, washed with DMAc (2 ml×5) and anhydrous acetone (2 ml×2), and dried at 100°C under vacuum, to produce corresponding X%AcTrz-COF-5 as grey solids in quantitative yield. Click reaction of 50%N 3 -COF-5 with other alkynes Alkyne compounds (4.03 mmol) (3-phenyl-1-propyne (500 μl), methyl propiolate (358 μl) or 1-hexyne (463 μl)) were added to a mixture of 50%N 3 -COF-5 (10 mg) and CuI (1.0 mg) in dry DMAc (1.0 ml) in Pyrex tube. The tube was degassed via three freeze–pump–thaw cycles, and the reaction mixture was stirred at 50°C for 24 h. The resulting precipitate was collected by centrifugation, washed with DMAc (2 ml×2) and anhydrous acetone (2 ml×5), and dried at 100°C under vacuum, to produce 50%RTrz-COF-5 as grey solids in quantitative yield. Click reaction for the synthesis of X%PyTrz-COF-5 PyMP (56.8 mg, 0.2 mmol) was added to an anhydrous DMAc (1.0 ml) suspension of X%N 3 -COF-5 ( X =5, 10 and 25) (10 mg) and CuI (1.5 mg) in Pyrex tube. The tube was degassed via three freeze–pump–thaw cycles, and the reaction mixture was stirred at 50°C for 24 h. The precipitate was collected by centrifugation, washed with DMAc (2 ml×5) and anhydrous acetone (2 ml×2), and dried at 100°C under vacuum, to produce X%PyTrz-COF-5 as a yellowish solid in quantitative yield. Synthesis of 100%N 3 -NiPc-COF A DMAc/ o -dichlorobenzene (2 ml/1 ml in volume) mixture of N 3 -BDBA (19.3 mg, 0.07 mmol) and (2,3,9,10,16,17,23,24-octahydroxyphthalocyanine) nickel(II) ([OH] 8 PcNi) (24.4 mg, 0.035 mmol) in a 10-ml Pyrex tube was degassed via three freeze–pump–thaw cycles. The tube was sealed and heated at 85°C for 7 days. The precipitate was collected by centrifugation, washed with anhydrous DMAc (2 ml×2) and anhydrous acetone (2 ml×5), and dried at 80°C under vacuum, to produce 100%N 3 -NiPc-COF as a deep green solid in 75% isolated yield. Click reaction for the synthesis of 100%EsTrz-NiPc-COF Methyl propiolate (358 ml) (4.03 mmol) was added to an anhydrous DMAc (1.0 ml) mixture of 100%N 3 -NiPc-COF (10 mg) and CuI (1.5 mg) in Pyrex tube. The tube was degassed via three freeze–pump–thaw cycles and the mixture was stirred at 50°C for 24 h. The precipitate was collected by centrifugation, washed with anhydrous DMAc (2 ml×2) and anhydrous acetone (2 ml×5), and dried at 100°C under vacuum, to produce 100%EsTrz-NiPc-COF as a deep green solid in quantitative yield. Characterization 1 H (400 MHz) and 13 C (100 MHz) NMR spectra were recorded on a JEOL JNM-LA400 spectrometer. FT IR spectra were recorded on a JASCO model FT IR-6100 infrared spectrometer, using KBr platelets. UV-VIS-IR diffuse reflectance spectrum (Kubelka–Munk spectrum) was recorded on a JASCO model V-670 spectrometer equipped with integration sphere model IJN-727. Fluorescence spectra of solid samples were recorded on a JASCO model FP-6600 spectrofluorometer. XRD data were recorded on a Rigaku model RINT Ultima III diffractometer, from 2 θ =1° up to 60° with 0.02° increment at 25°C. TGA measurements were carried out on a Mettler Toledo model TGA/SDTA 851e upon heating to 800°C at a rate constant of 10°C min –1 under nitrogen. Sorption measurements Nitrogen sorption was measured at 77 K with a Bel Japan Inc. model BELSORP-mini II analyser. Before measurement, the samples were degassed in vacuum at 150°C for more than 6 h. The BET method was utilized to calculate the specific surface areas. By using non-local density functional theory model, the pore volume and pore size distribution were derived a relative pressure P / P 0 <0.1. The calibration curve was obtained by using black carbon (Part No. 004-16833-00) as a reference material and nitrogen as an adsorption gas. CO 2 sorption was measured at 298 K using the same method as N 2 . Structure simulation Geometry optimization of the repeating unit was performed at B3LYP/6-31G(d) level by using the Gaussian 03 program package. The final molecular structure in a hexagonal unit cell was prepared by using geometrical parameters obtained from the optimized structure. Molecular modelling and Pawley refinement were carried out using Reflex, a software package for crystal determination from XRD pattern, implemented in MS modeling ver 4.4 (Accelrys Inc.) [38] , [39] . Unit-cell dimension was first manually determined from the observed XRD peak positions by using hexagonal arrangement. Using the obtained information, we performed Pawley refinement to optimize the lattice parameters iteratively until the R WP value converges. The refinement suggests a hexagonal crystal system with a unit cell of α = β =90° and γ =120°, a = b =30.01089 Å and c =3.45006 Å. The pseudo-Voigt profile function was used for whole-profile fitting, and Berrar–Baldinozzi function was used for asymmetry correction during the refinement processes. The final R WP and R P values were 7.50 and 4.79%, respectively. Simulated XRD patterns were calculated from this refined unit cell and compared with the experimentally observed patterns. How to cite this article: Nagai, A. et al . Pore surface engineering in covalent organic frameworks. Nat. Commun. 2:536 doi: 10.1038/ncomms1542 (2011).